Driving chemical reactions with polariton condensates 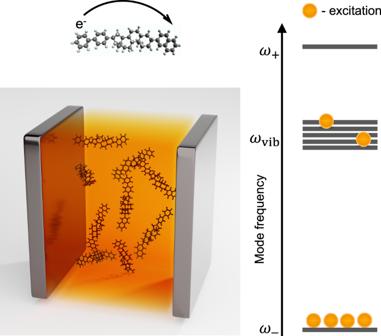Fig. 1: Vibrational polariton condensate. A large number of molecules are placed inside an optical cavity where their vibrations strongly couple to the cavity mode. The system is constantly pumped to create a polariton condensate and the right side of the figure depicts the occupation of different modes under condensation (frequencies of the upper polariton, dark modes, and lower polariton areω+,ωvib, andω−, respectively). The rate of intramolecular electron transfer under vibrational polariton condensation is investigated. When molecular transitions strongly couple to photon modes, they form hybrid light-matter modes called polaritons. Collective vibrational strong coupling is a promising avenue for control of chemistry, but this can be deterred by the large number of quasi-degenerate dark modes. The macroscopic occupation of a single polariton mode by excitations, as observed in Bose-Einstein condensation, offers promise for overcoming this issue. Here we theoretically investigate the effect of vibrational polariton condensation on the kinetics of electron transfer processes. Compared with excitation with infrared laser sources, the vibrational polariton condensate changes the reaction yield significantly at room temperature due to additional channels with reduced activation barriers resulting from the large accumulation of energy in the lower polariton, and the many modes available for energy redistribution during the reaction. Our results offer tantalizing opportunities to use condensates for driving chemical reactions, kinetically bypassing usual constraints of fast intramolecular vibrational redistribution in condensed phase. Light and matter couple strongly when a large number of molecules are placed within optical cavities that confine light [1] , [2] , [3] . As a result, hybrid light-matter excitations called polaritons form when a collective molecular transition and a photon mode coherently exchange energy faster than the individual decay from each component. Light-matter strong coupling (SC) opens up a new path to modify material properties by controlling their electromagnetic environment [4] , [5] . For instance, vibrational strong coupling (VSC), where an infrared cavity mode couples to an ensemble of localized molecular vibrations in a film or solution, influences chemical reactivity even without external pumping [6] , [7] . However, the microscopic mechanism for modification of molecular processes through hybridization with light is still poorly understood [8] , [9] , [10] , since it could be limited by the presence of a large number of quasi-degenerate dark modes that do not possess any photonic character and are likely to behave similarly to uncoupled molecules [10] . A Bose–Einstein condensate of polaritons [11] offers a solution to this problem since the macroscopic occupation of polaritonic states enhances the effects from SC. In the last decade, Bose–Einstein condensation has been demonstrated in several organic exciton-polariton systems at room temperature [12] , [13] , [14] , [15] . Recently, organic polariton condensates were used to build polariton transistors [16] , and theoretical predictions suggest they may also modify incoherent charge transport [17] . Interestingly, the consequences of polariton condensation on chemical reactivity have not been addressed in the literature prior to the present study. Ideas of using Bose–Einstein condensates of molecules in chemistry have been previously proposed, but they require ultracold temperatures due to the large mass of the condensing entities [18] , [19] . The low effective mass that polaritons inherit from their photonic component, along with the large binding energy of Frenkel excitons, enables room-temperature condensation [20] . The partly photonic character of polaritons also offers additional benefits such as delocalization and remote action for manipulating chemistry [21] . Here, we investigate the effect of polariton condensation on electron transfer (ET) (Fig. 1 ). While the reaction yield under infrared laser excitation, without SC, already differs from that under thermal equilibrium conditions [22] , [23] , polariton condensation amplifies this difference by changing the activation barrier for the forward and backward reactions unevenly, tilting the equilibrium towards either reactants or products. Fig. 1: Vibrational polariton condensate. A large number of molecules are placed inside an optical cavity where their vibrations strongly couple to the cavity mode. The system is constantly pumped to create a polariton condensate and the right side of the figure depicts the occupation of different modes under condensation (frequencies of the upper polariton, dark modes, and lower polariton are ω + , ω vib , and ω − , respectively). The rate of intramolecular electron transfer under vibrational polariton condensation is investigated. Full size image Bose–Einstein condensation of vibrational polaritons Bose–Einstein condensation of vibrational polaritons has not been experimentally achieved yet; however, as we shall argue, there are compelling reasons to believe that they are presently within reach. Most theoretical investigations on polariton condensation with organic microcavities involve systems under electronic strong coupling (ESC) [24] , [25] ; polariton condensation under VSC requires a separate treatment due to the difference in energy scales and the involved relaxation pathways [26] . While typical bare exciton energies range from 2–3 eV with Rabi splitting ~200 meV under ESC, the bare frequency of vibrations is 100–300 meV with Rabi splitting ~20−40 meV under VSC. Since the Rabi splitting is of the order of k B T at room temperature, thermal effects are crucial for vibrational polaritons. Under ESC, polariton relaxation is assisted by high-frequency intramolecular vibrations [27] , whereas, under VSC, low-frequency solvent modes play a key role in this process [28] , [29] , similar to what happens in THz phonon Fröhlich condensation in biomolecules [30] , [31] . We model the polariton system as a set of N vibrational modes ( \({\hat{a}}_{{{{{{{{\rm{vib}}}}}}}},j}\) ), with frequency ω vib , strongly coupled to a single photon mode ( \({\hat{a}}_{{{{{{{{\rm{ph}}}}}}}}}\) ) with frequency ω ph . In the Hamiltonian of the system, 
    Ĥ=	  ℏω_ph(â_ph^†â_ph+1/2)+ℏω_vib∑_j=1^N(â_vib,j^†â_vib,j+1/2)
     	+∑_j = 1^Nℏ g(â_vib,j^†â_ph+â_ph^†â_vib,j),
 (1) we have applied the rotating wave approximation. Upon diagonalizing this Hamiltonian, we get normal modes: lower and upper polaritons, and N − 1 dark mode with frequencies ω − , ω + , and \({\omega }_{{{{{{{{\rm{D}}}}}}}}}^{k}\) , respectively: 
    ω_± 	=ω_vib+Δ±Ω/2,
    ω_D^k 	=ω_vib         2≤ k≤ N,
 (2) where \({{\Omega }}=\sqrt{{{{\Delta }}}^{2}+4{g}^{2}N}\) is the Rabi splitting and Δ = ω ph − ω vib the detuning between cavity and molecular vibrations. To model polariton population dynamics, we use Boltzmann rate equations where the polariton system is weakly coupled to a low-frequency solvent bath, which enables scattering between modes [32] . These rate equations also account for final-state stimulation, 
    dn_i/dt=∑_j(W_ijn_j(1+n_i)-W_ji(1+n_j)n_i)-γ_in_i+P_i,
 (3) where n i is the population, γ i is the decay rate and P i is the external pumping rate of the i th mode. The scattering rate from mode j to i , W i j , satisfies detailed balance: \({W}_{ij}/{W}_{ji}={e}^{-\beta ({\epsilon }_{i}-{\epsilon }_{j})}\) . Here, β = 1/( k B T ), k B is the Boltzmann constant, T is the temperature, and ϵ i = ℏ ω i where ω i is the frequency of the i t h mode. The decay from different modes is \({\gamma }_{i}=| {c}_{{{{{{{{\rm{vib}}}}}}}}}^{i}{| }^{2}{{{\Gamma }}}_{\downarrow }+| {c}_{{{{{{{{\rm{ph}}}}}}}}}^{i}{| }^{2}\kappa\) , where \(| {c}_{{{{{{{{\rm{vib}}}}}}}}}^{i}{| }^{2}\) and \(| {c}_{{{{{{{{\rm{ph}}}}}}}}}^{i}{| }^{2}\) are the molecular and photon fraction, respectively, Γ ↓ is the decay rate of the molecular vibrations, and κ is the cavity leakage rate. Two factors play a determining role in the condensation threshold: (i) the rate of scattering between polariton and dark modes relative to losses from the system, i.e., the rate of thermalization and (ii) the abundance of modes close in energy to the condensing mode [33] . For all calculations, we assume fast thermalization. As mentioned in (ii), the presence of many modes close to the lower polariton would deter condensation by distributing the energy pumped into the system among all these modes. Thus, the energetic proximity between the dark state manifold, which has a large density of states (DOS), and the lower polariton pose one of the biggest challenges for polariton condensation under VSC. The distribution of excitations between the polariton and dark modes is shown in Fig. 2 for different detunings and we observe a condensation transition at ℏ Δ ≈ −1.5 k B T (see Supplementary Note 2 for details). Above the condensation threshold, a large fraction of excitations resides in the lower polariton \(\frac{{n}_{-}}{(\mathop{\sum }\nolimits_{k = 2}^{\infty }{n}_{{{{{{{{\rm{D}}}}}}}}}^{k})}\gg \frac{1}{(N-1){e}^{-\beta \hslash ({{\Omega }}-{{\Delta }})/2}}\) . Fig. 2: Polariton condensation transition. Fraction of excitations in different modes as a function of cavity detuning ℏ Δ = ℏ ω ph − ℏ ω vib while keeping the pumping rate P − fixed. The black curve includes the excitations in all dark modes taken together while the green and orange curves show the fraction excitations in the lower and upper polariton, respectively. The condensation transition takes place close to ℏ Δ ≈ −1.5 k B T . Here, the lower polariton is pumped with rate P − = 0.16 N Γ ↓ , the light-matter coupling \(2\hslash g\sqrt{N}=0.72{k}_{{{{{{{{\rm{B}}}}}}}}}T\) , the temperature k B T = 0.1389 ℏ ω vib ( T = 298 K when ℏ ω vib = 185 meV), number of molecules N = 10 7 and cavity leakage rate κ = Γ ↓ . Full size image The average population per molecule at the condensation threshold \(\bar{n}={P}_{{{{{{{{\rm{th}}}}}}}}}/N{{{\Gamma }}}_{\downarrow }\) is a good measure of the feasibility of vibrational polariton condensation. For instance, demanding population inversion, \(\bar{n} \, > \, 0.5\) , would be experimentally difficult to achieve in general. In Fig. 3 , we plot \(\bar{n}\) for different light-matter coupling strengths, \(2\hslash g\sqrt{N}\) , and detunings, ℏ Δ. Here, we numerically obtain P th as the pumping rate when 10% of the excitations are in the lower polariton. The threshold obtained this way closely corresponds with the theoretical condition for condensation 
    n̅_D^k  >  n_solvent(ℏ (Ω-Δ)/2),
 (4) where, \({\bar{n}}_{{{{{{{{\rm{D}}}}}}}}}^{k}=\frac{1}{N-1}\mathop{\sum }\nolimits_{k = 2}^{N}{n}_{{{{{{{{\rm{D}}}}}}}}}^{k}\) is the average occupation of a dark mode, and n solvent ( E ) is the Bose–Einstein population of a solvent mode with energy E at room temperature T room [33] . The energy difference between the lower polariton and the dark state reservoir ℏ (Ω − Δ)/2 determines the condensation threshold. From Fig. 3 we see that vibrational polariton condensation is feasible for water even at room temperature for up to zero detuning. Fig. 3: Polariton condensation threshold. Numerically obtained average population per molecule at the condensation threshold \(\bar{n}={P}_{{{{{{{{\rm{th}}}}}}}}}/N{{{\Gamma }}}_{\downarrow }\) (10% of the excitations are in the lower polariton), for a range of light-matter coupling strengths \(2\hslash g\sqrt{N}\) and cavity detunings ℏ Δ = ℏ ω ph − ℏ ω vib . In the black and purple regions of the plot (Δ > 0 and \(2\hslash g\sqrt{N}/{k}_{{{{{{{{\rm{B}}}}}}}}}T \, < \, 2\) ), the threshold for condensation is high, \(\bar{n}\gg 1\) , and polariton condensation is difficult to achieve experimentally. The threshold for condensation is much lower, \(\bar{n} \, < \, 0.1\) , for the lighter colored (yellow, orange) regions. In our plot above only the upper polariton is pumped and we use cavity leakage rate κ = Γ ↓ . The vertical lines correspond to \(2\hslash g\sqrt{N}/{k}_{{{{{{{{\rm{B}}}}}}}}}T\) at room temperature for H 2 O ( \(2\hslash g\sqrt{N}\approx 700{{{{{{{{\rm{cm}}}}}}}}}^{-1}\) ) and W(CO) 6 ( \(2\hslash g\sqrt{N}\approx 50{{{{{{{{\rm{cm}}}}}}}}}^{-1}\) ). Calculations in Figs. 4 – 6 are presented for the conditions in point A. Full size image Our model does not include disorder; as a result, all dark modes are degenerate at frequency ω vib , but in experimental systems, inhomogeneous broadening of transitions can lead to a nonzero density of dark states even at the bottom of the lower polariton branch [34] . This fact will affect the condensation threshold and should be considered in the future while looking for experimental systems that can demonstrate vibrational polariton condensation. Stimulating the lower polariton directly by shining a resonant laser on it [16] or using a Raman scattering scheme [35] can help overcome this issue by dynamically lowering the condensation threshold. Chemical reactions and vibrational polariton condensation Electron transfer has been theoretically studied under both ESC [36] , [37] and VSC [38] , [39] . Here, we look at how vibrational polariton condensation affects the rate of intramolecular nonadiabatic electron transfer using the VSC version [38] of the Marcus–Levich–Jortner (MLJ) model [40] , [41] , [42] . Our system consists of N molecules placed inside an optical cavity supporting a single photon mode with a bosonic operator \({\hat{a}}_{{{{{{{{\rm{ph}}}}}}}}}\) and frequency ω ph . The molecules can be in the reactant R or product P electronic state; for the i th molecule, these states are denoted by \(\left|{{{{{{{{\rm{R}}}}}}}}}_{i}\right\rangle\) and \(\left|{{{{{{{{\rm{P}}}}}}}}}_{i}\right\rangle\) , respectively. Each electronic state is dressed with a high-frequency intramolecular vibrational mode with a bosonic operator \({\hat{a}}_{x,i}\) and frequency ω vib where x = R, P; this mode couples to the photon mode. The equilibrium geometry of this vibrational mode depends on the electronic state according to, 
    â_R,i=D̂_i^†â_P,iD̂_i,
 (5) where \({\hat{D}}_{i}=\exp (({\hat{a}}_{{{{{{{{\rm{P}}}}}}}},i}^{{{{\dagger}}} }-{\hat{a}}_{{{{{{{{\rm{P}}}}}}}},i})\sqrt{S})\) and S is the Huang–Rhys factor. Apart from the intramolecular vibrations, an effective low-frequency solvent mode surrounding each molecule facilitates ET. It is treated classically, with q S, i and p S, i being its position and momentum. The Hamiltonian \(\hat{H}\) for the full system is a generalization of Eq. ( 1 ) to account for the chemical reaction, 
    Ĥ=Ĥ_0+V̂_react,
 (6) and 
    Ĥ_0	=Ĥ_ph+∑_i=1^N∑_x=R,P(Ĥ_x,i+V̂_x,i)|x_i⟩⟨x_i|,
    V̂_react	=∑_i=1^NJ_RP(|R_i⟩⟨P_i|+|P_i⟩⟨R_i|). (7) where \({\hat{H}}_{0}\) describes the photon ( \({\hat{H}}_{{{{{{{{\rm{ph}}}}}}}}}\) ), intramolecular vibrations and solvent modes of the i th molecule ( \({\hat{H}}_{x,i}\) ), and light-matter couplings ( \({\hat{V}}_{x,i}\) ). The diabatic coupling \({\hat{V}}_{{{{{{{{\rm{react}}}}}}}}}\) is a perturbation that couples R and P electronic states with coupling strength J RP . We have taken the dipole moment to be zero when the vibrational coordinate is in its equilibrium position in both R and P electronic states. Relaxing this assumption will add terms of the form \({c}_{x}({\hat{a}}_{{{{{{{{\rm{ph}}}}}}}}}+{\hat{a}}_{{{{{{{{\rm{ph}}}}}}}}})\left|{x}_{i}\right\rangle \left\langle {x}_{i}\right|\) to the Hamiltonian and will not affect the reaction rates calculated. Ĥ_ph 	=ℏω_ph(â_ph^†â_ph+1/2),
    Ĥ_R,i 	=ℏω_vib(â_R,i^†â_R,i+1/2)+1/2ℏω_S(| p_S,i| ^2+| q_S,i+d_S| ^2),
    Ĥ_P,i 	=ℏω_vib(â_P,i^†â_P,i+1/2)+1/2ℏω_S(| p_S,i| ^2+| q_S,i| ^2)+ΔG,
    V̂_x,i 	=ℏg_x(â_x,i^†â_ph+â_ph^†â_x,i),
 (8) where Δ G is the free-energy difference of each individual molecule reaction. We construct potential energy surfaces (PES) by parametrically diagonalizing \({\hat{H}}_{0}\) as a function of the solvent coordinate q S, i . The operators \({\hat{N}}_{{{{{{{{\rm{R}}}}}}}}}=\mathop{\sum }\nolimits_{i = 1}^{N}\left|{{{{{{{{\rm{R}}}}}}}}}_{i}\right\rangle \left\langle {{{{{{{{\rm{R}}}}}}}}}_{i}\right|\) and \({\hat{N}}_{{{{{{{{\rm{P}}}}}}}}}=\mathop{\sum }\nolimits_{i = 1}^{N}\left|{{{{{{{{\rm{P}}}}}}}}}_{i}\right\rangle \left\langle {{{{{{{{\rm{P}}}}}}}}}_{i}\right|\) commute with H 0 and correspond to the number of R and P molecules, respectively. While dynamics under \({\hat{H}}_{0}\) conserves N R , N P , the effect of \({\hat{V}}_{{{{{{{{\rm{react}}}}}}}}}\) is to induce reactive transitions that modify those quantities while keeping N = N R + N P constant. We assign the label 1 ≤ i ≤ N R to R molecules, and N R + 1 ≤ i ≤ N to P molecules. We also reorganize the intramolecular vibrations into a single bright mode, 
    â_B(N_R,N_P)=1/√(g_R^2N_R+g_P^2N_P)(g_R∑_i=1^N_Râ_R,i+g_P∑_i=N_R+1^Nâ_P,i),
 (9) that possesses the correct symmetry to couple with light and N − 1 dark modes (D k ), 
    â_D(N_R,N_P)^k=∑_i=1^N_Rc_k,iâ_R,i+∑_i=N_R+1^Nc_k,iâ_P,i,
 (10) labeled by an additional index 2 ≤ k ≤ N , which do not couple with light. The dark modes are orthogonal to the bright mode \({g}_{{{{{{{{\rm{R}}}}}}}}}\mathop{\sum }\nolimits_{i = 1}^{{N}_{{{{{{{{\rm{R}}}}}}}}}}{c}_{k,i}+{g}_{{{{{{{{\rm{P}}}}}}}}}\mathop{\sum }\nolimits_{i = {N}_{{{{{{{{\rm{R}}}}}}}}}+1}^{N}{c}_{k,i}=0\) , and to each other \(\mathop{\sum }\nolimits_{i = 1}^{N}{c}_{k,i}{c}_{k^{\prime} ,i}^{* }={\delta }_{k,k^{\prime} }\) . Unless mentioned otherwise, the number of R and P molecules is N R and N P , respectively, and for brevity, we will drop ( N R , N P ) dependence in the subscript. The bright and photon modes combine to form the upper polariton (UP) \({\hat{a}}_{+}\) , and lower polariton (LP) \({\hat{a}}_{-}\) , modes: 
    â_+	=cosθâ_ph+sinθâ_B,
    â_-	=sinθâ_ph-cosθâ_B,
 (11) with mixing angle, 
    θ =tan^-1[Ω-Δ/2√(g_R^2N_R+g_P^2N_P)],
 (12) where \({{\Omega }}=\sqrt{{{{\Delta }}}^{2}+4({g}_{{{{{{{{\rm{R}}}}}}}}}^{2}{N}_{{{{{{{{\rm{R}}}}}}}}}+{g}_{{{{{{{{\rm{P}}}}}}}}}^{2}{N}_{{{{{{{{\rm{P}}}}}}}}})}\) is the Rabi splitting, and Δ = ω ph − ω vib the detuning between the cavity and molecular vibrations. The eigenstates of \({\hat{H}}_{0}\) are the dark, upper, and lower polariton modes with frequencies given in Eq. ( 2 ). According to the MLJ theory, the rate constant for ET outside of an optical cavity depends on properties of the intramolecular and solvent modes [40] , [41] , [42] . Under laser driving, this rate constant is, 
    k_R→P^IR=∑_n=0^∞P_n̅(n)k_R→P(n)
 (13) where 
    k_R→P(n) 	=√(π/λ_Sk_BT)| J_RP| ^2/ℏ∑_f=-n^∞| ⟨ n| n+f⟩ ^'| ^2exp(-E_f^/k_BT),
    P_n̅(n) 	=e^-n̅n̅^n/n!,
    E_f^ 	=(ΔG+λ_S+fℏω_vib)^2/4λ_S,
    ⟨ n| n+f⟩ ^' 	=⟨ n|D̂_i|n+f⟩ . (14) Here, \({P}_{\bar{n}}(n)\) is the Poisson distribution with average mode population \(\bar{n}\) , λ S is the solvent reorganization energy, \({E}_{f}^{{{{\ddagger}}} }\) is the activation energy, and \(| \left\langle n| n+f\right\rangle ^{\prime} {| }^{2}\) is the Franck–Condon (FC) factor, where \(\left|n\right\rangle\) and \(\left|n+f\right\rangle ^{\prime}\) are the intramolecular initial and final states, respectively. \({P}_{\bar{n}}(n)\) has been taken to correspond to the ideal laser-driven-damped harmonic oscillator, leading to a coherent state in the vibrational mode. The presence of anharmonic couplings would lead to intramolecular vibrational energy redistribution (IVR) [43] , reducing the value of \({P}_{\bar{n}}(n)\) for high-lying Fock states. 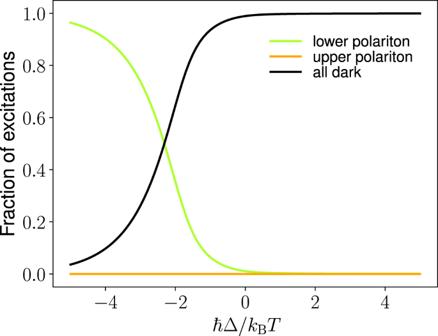Fig. 2: Polariton condensation transition. Fraction of excitations in different modes as a function of cavity detuningℏΔ =ℏωph−ℏωvibwhile keeping the pumping rateP−fixed. The black curve includes the excitations in all dark modes taken together while the green and orange curves show the fraction excitations in the lower and upper polariton, respectively. The condensation transition takes place close toℏΔ ≈ −1.5kBT. Here, the lower polariton is pumped with rateP−= 0.16NΓ↓, the light-matter coupling\(2\hslash g\sqrt{N}=0.72{k}_{{{{{{{{\rm{B}}}}}}}}}T\), the temperaturekBT= 0.1389ℏωvib(T= 298 K whenℏωvib= 185 meV), number of moleculesN= 107and cavity leakage rateκ= Γ↓. However, as we shall see below, even under these ideal circumstances, the condensate can outcompete the laser-driven situation in terms of reactivity. We thus expect the benefits of the condensate to be enhanced when IVR processes are taken into account. Apart from vibrations within the reacting molecule, under VSC, the ET process also depends on vibrations in all other molecules and the photon mode, and can be represented by, 
    ∑_k=2^ND_k+LP+UP→∑_k=2^ND_k^' +LP^' +UP^' . (15) Here and hereafter, the primed and unprimed quantities refer to electronic states with ( N R , N P ) and ( N R − 1, N P + 1) reactant-product distributions, respectively. The symmetry of the light-matter coupling allows us to use the dark state basis introduced in [44] and [38] to reduce the number of modes involved in the reaction from N + 1 to three, 
    D_R,c+LP+UP→D_P,c^' +LP^' +UP^' . (16) Here, the c th molecule is reacting, while D x , c and \({{{{{{{{\rm{D}}}}}}}}_{x,c}^{\prime}}\) are dark modes highly localized in it, with corresponding operators \({\hat{a}}_{{{{{{{{\rm{D}}}}}}}}}^{(R,c)}\) and \({\hat{a}}_{{{{{{{{\rm{D}}}}}}}}}^{(P,c)^{\prime} }\) (see Supplementary Note 1 ). We perform all our calculations in this subsection using parameters from point A in Fig. 3 but while pumping the lower polariton. Here, ℏ Δ = −0.5 k B T , \(2\hslash g\sqrt{N}=0.72{k}_{{{{{{{{\rm{B}}}}}}}}}T\) , k B T = 0.1389 ℏ ω vib ( T = 298 K when ℏ ω vib = 185 meV) and N = 10 7 ; we choose pumping rate P − = 0.08 N Γ ↓ , which leads to average mode populations N + = 0.064, N − = 1.94 × 10 4 and N D = 0.078 under symmetric coupling g R = g P = g . Here, 2.4% of all excitations reside in the lower polariton. To compare the reaction rates under polariton condensation and outside the cavity under pumping, we take \(\bar{n}=0.08\) in Eq. ( 13 ). Under condensation, the initial vibrational state of the system can be described by \(\rho ={\sum }_{{n}_{+},{n}_{-},{n}_{{{{{{{{\rm{D}}}}}}}}}}P({n}_{+},{n}_{-},{n}_{{{{{{{{\rm{D}}}}}}}}})\left|{n}_{+},{n}_{-},{n}_{{{{{{{{\rm{D}}}}}}}}}\right\rangle \left\langle {n}_{+},{n}_{-},{n}_{{{{{{{{\rm{D}}}}}}}}}\right|\) , where the entries in \(\left|{n}_{+},{n}_{-},{n}_{{{{{{{{\rm{D}}}}}}}}}\right\rangle\) label number of quanta in the UP, LP, and D R, c modes, respectively. The results from the rate equations Eq. ( 3 ) provide us only with the average steady-state mode populations, N + , N − , and N D , and not the distribution P ( n + , n − , n D ). For simplicity, we assume the semiclassical approximation \(P({n}_{+},{n}_{-},{n}_{{{{{{{{\rm{D}}}}}}}}})\approx {\delta }_{{n}_{+},0}{P}_{{N}_{{{{{{{{\rm{D}}}}}}}}}}^{{{{{{{{\rm{th}}}}}}}}}({n}_{{{{{{{{\rm{D}}}}}}}}}){\delta }_{{n}_{-},{N}_{-}}\) , where \({P}_{{N}_{{{{{{{{\rm{D}}}}}}}}}}^{{{{{{{{\rm{th}}}}}}}}}(n)\) is the thermal distribution with average population N D . This approximation is reasonable for populations N + < N D ≪ 1 ≪ N − , 
    ρ =∑_n_DP_N_D^th(n_D)|0,N_-,n_D⟩⟨ 0,N_-,n_D|. (17) The product vibrational states are \(\left|{\nu }_{+},{\nu }_{-},{\nu }_{{{{{{{{\rm{D}}}}}}}}}\right\rangle ^{\prime}\) . We assume that cavity leakage and the rate of scattering between modes is much faster than the rate of the chemical reaction. For a cavity with ~100 ps lifetime and ET reactions with 1/ k R→P ~ 10 6 − 10 2 ps [45] , this assumption is valid. Therefore, if the populations of polariton modes change during the course of the reaction, they quickly reach a steady state before the next molecule reacts. Similarly, we also assume that the polariton and dark mode populations reach a steady state before the backward reaction takes place while computing the rate constant \({k}_{{{{{{{{\rm{P}}}}}}}}\to {{{{{{{\rm{R}}}}}}}}}^{{{{{{{{\rm{cond}}}}}}}}}\) . Generalizing the cavity MLJ theory presented in ref. [38] , we calculate the rate constant 
    k_R→P^cond=∑_n=0^∞P_N_D^th(n)k_R→P^cond(n)
 (18) for the forward reaction under polariton condensation, where 
    k_R→P^cond(n)=	  √(π/λ_Sk_BT)| J_RP| ^2/ℏ∑_ν_+=0^∞∑_ν_-=0^∞∑_ν_D=0^∞W_ν_+,ν_-,ν_D^f,n,
    W_ν_+,ν_-,ν_D^f,n=	  | F_ν_+,ν_-,ν_D^f,n| ^2×exp(-E_ν_+,ν_-,ν_D^f,n/k_BT). (19) The FC factor \(| {F}_{{\nu }_{+},{\nu }_{-},{\nu }_{{{{{{{{\rm{D}}}}}}}}}}^{f,n}{| }^{2}=\big| \left\langle 0,{N}_{-},n| {\nu }_{+},{\nu }_{-},{\nu }_{{{{{{{{\rm{D}}}}}}}}}\right\rangle ^{\prime}\big| ^{2}\) , and activation energy \({E}_{{\nu }_{+},{\nu }_{-},{\nu }_{{{{{{{{\rm{D}}}}}}}}}}^{f,n{{{\ddagger}}} }\) play an important role in determining the rate constant. While many methods have been developed for computing multimode FC factors [46] , [47] , [48] , the focus has been on increasing the number of modes while keeping their occupation small. The current problem, however, offers a new technical challenge: the large occupation of LP makes the aforementioned methods computationally expensive. Instead, we draw inspiration from previous work that employs generating functions [47] and combine those techniques with the powerful Lagrange–Bürmann formula [49] to obtain analytical expressions for the required three-dimensional FC factors (see details in Supplementary Section S3 ). The activation energies for the various channels of reactivity are, 
    E_ν_+,ν_-,ν_D^f,n=(E_P^ν_+,ν_-,ν_D-E_R^0,N_-,n+λ_S)^2/4λ_S,
 (20) where 
    E_P^ν_+,ν_-,ν_D=	  ΔG+ℏ[ω_+^'(ν_++1/2). .+ ω_-^'(ν_-+1/2)+ω_vib(ν_D+1/2)],
    E_R^0,N_-,n=	  ℏ[ω_+1/2+ω_-(N_-+1/2)+ω_vib(n+1/2)]. (21) When condensation takes place, the number of quanta in the lower polariton N − ~10 5 is so large that the summation in \({k}_{{{{{{{{\rm{R}}}}}}}}\to {{{{{{{\rm{P}}}}}}}}}^{{{{{{{{\rm{cond}}}}}}}}}(n)\) becomes difficult to estimate. To simplify the computation and gain intuition, we group channels into sets with the same change in the total number of intramolecular vibrational quanta f = ν + + ν − + ν D − N − − n upon ET. The closeness in energy between PES with the same f , and hence similar activation barriers, is the rationale for this grouping. \({k}_{{{{{{{{\rm{R}}}}}}}}\to {{{{{{{\rm{P}}}}}}}}}^{{{{{{{{\rm{cond}}}}}}}}}(n)\) then goes from a free summation over three indices ν + , ν − and ν D into a summation over four indices f , ν + , ν − and ν D with the constraint ν + + ν − + ν D = N − + n + f , 
    k_R→P^cond(n)=	  √(π/λ_Sk_BT)| J_RP| ^2/ℏ
    ∑_f=-N_--n^∞∑_ν_+,ν_-,ν_D^ν_++ν_-+ν_D=N_-+n+fW_ν_+,ν_-,ν_D^f,n. (22) To understand the qualitative difference between reactions under polariton condensation and external pumping without SC, in Fig. 4 a, b we plot the PESs (not to scale) showing the forward reaction under symmetric light-matter coupling and zero detuning. The yellow (black) parabolas in Fig. 4 a, b represent PESs for a molecule in the electronic state \(\left|{{{{{{{\rm{R}}}}}}}}\right\rangle\) ( \(\left|{{{{{{{\rm{P}}}}}}}}\right\rangle\) ) and vibrational state \(\left|2\right\rangle\) ( \(\left|2+f\right\rangle ^{\prime}\) ) in Fig. 4 a and \(\left|0,{N}_{-},2\right\rangle\) ( \(\left|0,{N}_{-},2+f\right\rangle ^{\prime}\) ) in Fig. 4 b. The red parabolas in Fig. 4 b are additional final PESs provided by the vibrational polariton condensate (hereafter referred to solely as “condensate”) that account for all other final vibrational states \(\left|{\nu }_{+},{\nu }_{-},{\nu }_{{{{{{{{\rm{D}}}}}}}}}\right\rangle ^{\prime}\) . Fig. 4: Potential energy surfaces (not to scale) and reaction yield. a , c , e are results for a laser-driven system without light-matter strong coupling (SC) and b , d , f are for the same system under SC and 2.4% of the population in the lower polariton (condensation). All these plots are for symmetric light-matter coupling g R = g P . a , b For a clearer qualitative picture, we plot the PESs under zero detuning Δ = 0. Initial (yellow) and final (black) PESs for a molecule undergoing the forward reaction with solvent coordinate q S,c . While the energy separation between black PESs is ℏ ω vib , the condensate provides many additional final PESs (red, separated by ℏ Ω/2 at resonance). c Reaction yield \({N}_{{{{{{{{\rm{P}}}}}}}}}^{{{{{{{{\rm{ss}}}}}}}}}/N\) at temperature k B T = 0.1389 ℏ ω vib ( T = 298 K when ℏ ω vib = 185 meV), Huang–Rhys factor S = 3.5, and average occupation of the intramolecular vibrational mode \(\bar{n}=0.08\) . d Reaction yield \({N}_{{{{{{{{\rm{P}}}}}}}}}^{{{{{{{{\rm{ss}}}}}}}}}/N\) with Δ = − 0.0695 ω vib , \(2{g}_{{{{{{{{\rm{R}}}}}}}}}\sqrt{N}=2{g}_{{{{{{{{\rm{P}}}}}}}}}\sqrt{N}=0.1{\omega }_{{{{{{{{\rm{vib}}}}}}}}}\) , P − = 0.08 N Γ ↓ , N = 10 7 , temperature and Huang–Rhys factor are the same as c . The contributions of the red PESs through the condensate provide a broader tunability of reaction yields with respect to Δ G than under laser driving without SC. Notice that originally endergonic (exergonic) reactions in the absence of optical pumping can become exergonic (endergonic) under the featured nonequilibrium conditions. e , f A cross-section of plot ( c , d ) when λ S = 10 −2 ℏ ω vib . The pink shaded regions correspond to cases where the dominant forward (backward) channel is in the inverted (normal) regime; the opposite is true for the green shaded regions. The condensate amplifies the forward (backward) reaction in the pink (green) shaded regions. Full size image The net rate of ET is, 
    dN_R/dt=-k_R→P^zN_R+k_P→R^zN_P,
 (23) where \({k}_{{{{{{{{\rm{R}}}}}}}}\to {{{{{{{\rm{P}}}}}}}}}^{z}\) and \({k}_{{{{{{{{\rm{P}}}}}}}}\to R}^{z}\) ( z = IR, cond) are the rate constants for the forward and backward reactions, respectively, which are themselves functions of N R and N P when g R ≠ g P . We find the steady-state solution \({N}_{{{{{{{{\rm{R}}}}}}}}}^{{{{{{{{\rm{ss}}}}}}}}}\) from this equation and compute the reaction yield \({N}_{{{{{{{{\rm{P}}}}}}}}}^{{{{{{{{\rm{ss}}}}}}}}}/N\) . The difference in yield between the condensate and bare case is particularly large when λ S ≪ ℏ ω vib < ∣ Δ G ∣ (see Fig. 4 c, d for symmetric coupling g R = g P ). To understand the underlying reason, we define the dominant channel \({f}_{\min }\) as the one with minimum activation barrier outside of the cavity. 1/k_BTdE_f^/df=ℏω_vib/k_BT(ΔG+λ_S+fℏω_vib/2λ_S)
 (24) Setting the derivative in Eq. ( 24 ) equal to zero and taking into account the discrete nature of f , we find the dominant channel, \({f}_{\min }=\left\lceil\frac{-{{\Delta }}G-{\lambda }_{{{{{{{{\rm{S}}}}}}}}}}{\hslash {\omega }_{{{{{{{{\rm{vib}}}}}}}}}}\right\rceil\) or \(\left\lfloor\frac{-{{\Delta }}G-{\lambda }_{{{{{{{{\rm{S}}}}}}}}}}{\hslash {\omega }_{{{{{{{{\rm{vib}}}}}}}}}}\right\rfloor\) . When λ S ≪ ℏ ω vib , ∣ Δ G ∣ , this channel contributes most to the rate constant because \(\frac{1}{{k}_{{{{{{{{\rm{B}}}}}}}}}T}\left|\frac{d{E}_{f}^{{{{\ddagger}}} }}{df}\right|\gg 1\) . We define Marcus normal \(\frac{d{E}_{f}^{{{{\ddagger}}} }}{df}{\Big|}_{{f}_{\min }} > \, 0\) and inverted \(\frac{d{E}_{f}^{{{{\ddagger}}} }}{df}{\Big|}_{{f}_{\min }} < \, 0\) regimes with respect to the dominant channel. If the dominant forward channel is in the inverted regime, the dominant backward channel (which can be found by replacing Δ G → − Δ G in Eq. ( 24 )) will be in the normal regime when λ S ≪ ℏ ω vib , ∣ Δ G ∣ . In Fig. 4 d, we see periodic yield modification in Δ G with period ~ ℏ ω vib , which decays for large Δ G / ℏ ω vib due to concomitant decline in FC factor for large changes in the number of vibrational quanta between the initial and final states. Outside of the cavity, we only see the first fringe (Fig. 4 c). To observe the full periodic structure in yield, we need a large occupation of higher vibrational states which requires very large pumping rates outside of the cavity. However, under polariton condensation, the macroscopic population of the lower polariton enables these interesting periodic features to be observed at room temperature with experimentally attainable pumping rates. Additionally, polariton condensation not only modifies the reaction yield under symmetric light-matter coupling strengths, as seen in Fig. 4 , it also changes the yield when the reactant and product asymmetrically couple with light (Fig. 5 ). Fig. 5: Reaction yield for asymmetric light-matter coupling. a , c The yield of the reaction when only the product (reactant) weakly couples with light. b , d Analogous plots under strong coupling \(2{g}_{{{{{{{{\rm{P}}}}}}}}}\sqrt{N}=0.1{\omega }_{{{{{{{{\rm{vib}}}}}}}}}\) , g R = 0 ( g P = 0, \(2{g}_{{{{{{{{\rm{R}}}}}}}}}\sqrt{N}=0.1{\omega }_{{{{{{{{\rm{vib}}}}}}}}}\) ). We use parameters Δ = −0.0695 ω vib , k B T = 0.1389 ℏ ω vib ( T = 298K when ℏ ω vib = 185 meV), S = 3.5, P − = 0.08 N Γ ↓ and N = 10 7 . We assume the same scattering parameters W i j and decay rates Γ ↓ , κ as in Fig. 2 . Full size image Condensation provides many additional channels for the forward and backward reactions (separated by ~ ℏ Ω/2, see red curves in Fig. 4 b, showing only the forward channels at resonance Δ = 0) due to transfer of quanta between the polariton and dark modes during the reaction. Condensation speeds up the reaction when the dominant channel is either in the inverted or in the normal regime (Fig. 6 b). This is the case because there are additional channels with energy both higher (benefiting the inverted regime) and lower (benefiting the normal regime) than the dominant channel (see red curves in Fig. 4 b). Apart from reduced activation energy, the additional channels provided by the condensate also have large enough FC factors to affect the rate constant. Reaction channels that involve changes in the number of quanta in the LP during the reaction have significantly larger FC factors (~10 20 times) under condensation N − = 0.1 N than without any pumping N − = 0 (Fig. S1 in the supplementary information compares them). 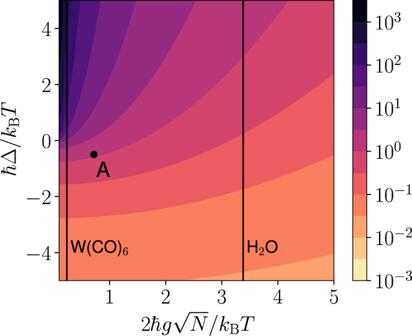Fig. 3: Polariton condensation threshold. Numerically obtained average population per molecule at the condensation threshold\(\bar{n}={P}_{{{{{{{{\rm{th}}}}}}}}}/N{{{\Gamma }}}_{\downarrow }\)(10% of the excitations are in the lower polariton), for a range of light-matter coupling strengths\(2\hslash g\sqrt{N}\)and cavity detuningsℏΔ =ℏωph−ℏωvib. In the black and purple regions of the plot (Δ > 0 and\(2\hslash g\sqrt{N}/{k}_{{{{{{{{\rm{B}}}}}}}}}T \, < \, 2\)), the threshold for condensation is high,\(\bar{n}\gg 1\), and polariton condensation is difficult to achieve experimentally. The threshold for condensation is much lower,\(\bar{n} \, < \, 0.1\), for the lighter colored (yellow, orange) regions. In our plot above only the upper polariton is pumped and we use cavity leakage rateκ= Γ↓. The vertical lines correspond to\(2\hslash g\sqrt{N}/{k}_{{{{{{{{\rm{B}}}}}}}}}T\)at room temperature for H2O (\(2\hslash g\sqrt{N}\approx 700{{{{{{{{\rm{cm}}}}}}}}}^{-1}\)) and W(CO)6(\(2\hslash g\sqrt{N}\approx 50{{{{{{{{\rm{cm}}}}}}}}}^{-1}\)). Calculations in Figs.4–6are presented for the conditions in point A. 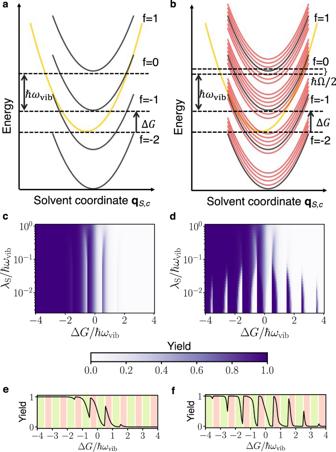Fig. 4: Potential energy surfaces (not to scale) and reaction yield. a,c,eare results for a laser-driven system without light-matter strong coupling (SC) andb,d,fare for the same system under SC and 2.4% of the population in the lower polariton (condensation). All these plots are for symmetric light-matter couplinggR=gP.a,bFor a clearer qualitative picture, we plot the PESs under zero detuning Δ = 0. Initial (yellow) and final (black) PESs for a molecule undergoing the forward reaction with solvent coordinateqS,c. While the energy separation between black PESs isℏωvib, the condensate provides many additional final PESs (red, separated byℏΩ/2 at resonance).cReaction yield\({N}_{{{{{{{{\rm{P}}}}}}}}}^{{{{{{{{\rm{ss}}}}}}}}}/N\)at temperaturekBT= 0.1389ℏωvib(T= 298 K whenℏωvib= 185 meV), Huang–Rhys factorS= 3.5, and average occupation of the intramolecular vibrational mode\(\bar{n}=0.08\).dReaction yield\({N}_{{{{{{{{\rm{P}}}}}}}}}^{{{{{{{{\rm{ss}}}}}}}}}/N\)with Δ = − 0.0695ωvib,\(2{g}_{{{{{{{{\rm{R}}}}}}}}}\sqrt{N}=2{g}_{{{{{{{{\rm{P}}}}}}}}}\sqrt{N}=0.1{\omega }_{{{{{{{{\rm{vib}}}}}}}}}\),P−= 0.08NΓ↓,N= 107, temperature and Huang–Rhys factor are the same asc. The contributions of the red PESs through the condensate provide a broader tunability of reaction yields with respect to ΔGthan under laser driving without SC. Notice that originally endergonic (exergonic) reactions in the absence of optical pumping can become exergonic (endergonic) under the featured nonequilibrium conditions.e,fA cross-section of plot (c,d) whenλS= 10−2ℏωvib. The pink shaded regions correspond to cases where the dominant forward (backward) channel is in the inverted (normal) regime; the opposite is true for the green shaded regions. The condensate amplifies the forward (backward) reaction in the pink (green) shaded regions. Changes in the rate constant as a function of λ S (Fig. 6 a) and Δ G (Fig. 6 b) are large for small λ S / ℏ ω vib and when Δ G / ℏ ω vib = n /2 where n is an odd integer since activation energy effects are large for these set of parameters. Fig. 6: Rate constant. Ratio of the rate constants inside \({k}_{{{{{{{{\rm{R}}}}}}}}\to {{{{{{{\rm{P}}}}}}}}}^{{{{{{{{\rm{cond}}}}}}}}}\) and outside \({k}_{{{{{{{{\rm{R}}}}}}}}\to {{{{{{{\rm{P}}}}}}}}}^{{{{{{{{\rm{IR}}}}}}}}}\) of the cavity under laser excitation with Δ = −0.0695 ω vib , k B T = 0.1389 ℏ ω vib ( T = 298 K when ℏ ω vib = 185 meV), S = 3.5, \(2g\sqrt{N}=0.1{\omega }_{{{{{{{{\rm{vib}}}}}}}}}\) , P − = 0.08 N Γ ↓ and N = 10 7 for symmetric coupling g R = g P = g . a Relative rate constant as a function of reorganization energy, λ S , with Δ G = −3.33 ℏ ω vib (the pink curve; here, the dominant channel lies in the inverted regime) and Δ G = −3.73 ℏ ω vib (the green curve; here, the dominant channel lies in the normal regime) and b as a function of Δ G with λ S = 10 −2 ℏ ω vib . Here, the pink region corresponds to the dominant channel in the inverted regime and the green to the normal regime. Full size image Our result is a first step towards understanding the effect of Bose–Einstein condensation of polaritons on chemical reactivity. We demonstrate this effect using a simple electron transfer model (MLJ) with molecular vibrations strongly coupled to light. In particular, we show that one can counteract the massive degeneracy of dark modes and enhance polaritonic effects by having a macroscopic occupation of the lower polariton mode i.e., Bose–Einstein condensation. Our results indicate that the latter is feasible for experimentally realizable pump powers and Rabi splittings, despite the close proximity in the energy of the dark state manifold with ℏ Ω ~ k B T . These results can guide the choice of suitable materials for condensation under VSC. While laser driving without SC modifies the reaction yield, this change is amplified by the condensate, due to the availability of many additional reactive channels that differ in energy by ~ ℏ Ω/2 rather than ~ ℏ ω vib . For a wide range of parameters, we find that this leads to a periodic dependence of reaction yield as a function of Δ G (with period ~ ℏ ω vib ), rendering a set of originally endergonic reactions exergonic, and vice versa. These effects are substantially weaker under laser driving and highlight both the energetic (availability of additional channels with lower activation energy) and entropic (redistribution of vibrational energy from the condensate into the polariton and dark modes upon reaction) advantages of exploiting polariton condensates for reactivity. 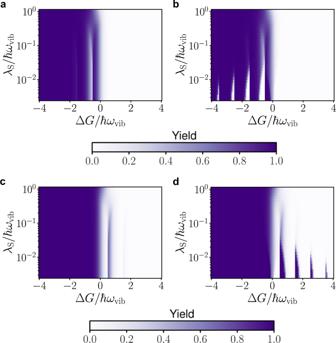Fig. 5: Reaction yield for asymmetric light-matter coupling. a,cThe yield of the reaction when only the product (reactant) weakly couples with light.b,dAnalogous plots under strong coupling\(2{g}_{{{{{{{{\rm{P}}}}}}}}}\sqrt{N}=0.1{\omega }_{{{{{{{{\rm{vib}}}}}}}}}\),gR= 0 (gP= 0,\(2{g}_{{{{{{{{\rm{R}}}}}}}}}\sqrt{N}=0.1{\omega }_{{{{{{{{\rm{vib}}}}}}}}}\)). We use parameters Δ = −0.0695ωvib,kBT= 0.1389ℏωvib(T= 298K whenℏωvib= 185 meV),S= 3.5,P−= 0.08NΓ↓andN= 107. We assume the same scattering parametersWijand decay rates Γ↓,κas in Fig.2. 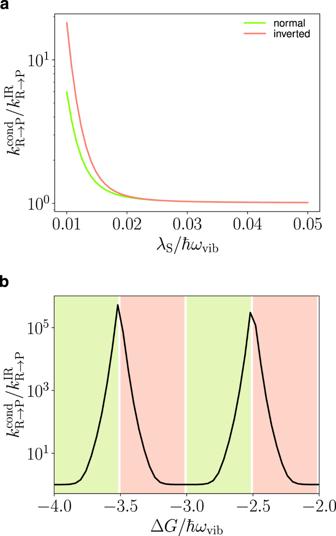Fig. 6: Rate constant. Ratio of the rate constants inside\({k}_{{{{{{{{\rm{R}}}}}}}}\to {{{{{{{\rm{P}}}}}}}}}^{{{{{{{{\rm{cond}}}}}}}}}\)and outside\({k}_{{{{{{{{\rm{R}}}}}}}}\to {{{{{{{\rm{P}}}}}}}}}^{{{{{{{{\rm{IR}}}}}}}}}\)of the cavity under laser excitation with Δ = −0.0695ωvib,kBT= 0.1389ℏωvib(T= 298 K whenℏωvib= 185 meV),S= 3.5,\(2g\sqrt{N}=0.1{\omega }_{{{{{{{{\rm{vib}}}}}}}}}\),P−= 0.08NΓ↓andN= 107for symmetric couplinggR=gP=g.aRelative rate constant as a function of reorganization energy,λS, with ΔG= −3.33ℏωvib(the pink curve; here, the dominant channel lies in the inverted regime) and ΔG= −3.73ℏωvib(the green curve; here, the dominant channel lies in the normal regime) andbas a function of ΔGwithλS= 10−2ℏωvib. Here, the pink region corresponds to the dominant channel in the inverted regime and the green to the normal regime. To summarize, vibrational polariton condensation offers a novel strategy to accumulate energy into a well-defined normal mode, a holy-grail in the field of vibrational dynamics that has been historically hindered by IVR. Its successful demonstration could revive hopes of “mode selective chemistry” [50] , beyond electron transfer processes. In future work, it will be interesting to explore how the studied phenomena generalize to molecular polariton condensates in different spectral ranges.